Polymeric pseudo-crown ether for cation recognition via cation template-assisted cyclopolymerization Cyclopolymerization is a chain polymerization of bifunctional monomers via alternating processes of intramolecular cyclization and intermolecular addition, to give soluble linear polymers consisting of in-chain cyclic structures. Though cyclopolymers comprising in-chain multiple large rings potentially show unique functionality, they generally require the elaborate design of bifunctional monomers. Here we report cation template-assisted cyclopolymerization of poly(ethylene glycol) dimethacrylates as an efficient strategy directly yielding polymeric pseudo-crown ethers with large in-chain cavities (up to 30-membered rings) for selective molecular recognition. The key is to select a size-fit metal cation for the spacer unit of the divinyl monomers to form a pseudo-cyclic conformation, where the two vinyl groups are suitably positioned for intramolecular cyclization. The marriage of supramolecular chemistry and polymer chemistry affords efficient, one-pot chemical transformation from common chemical reagents with simple templates to functional cyclopolymers. The marriage of supramolecular/organic chemistry and polymer chemistry is a promising strategy for the efficient and selective synthesis of designed materials [1] , [2] , [3] . It often involves template molecules that non-covalently or covalently interact with substrates, to induce a specific conformation, in which reactive sites and substrates are oriented suitably for chemical bond formation. For example, such a template-directed synthesis [4] , [5] , [6] , [7] , [8] , [9] , [10] utilizing supramolecular interaction or molecular recognition is quite effective for intramolecular cyclization by bringing reactive sites close to one another. Metal (M + ) or ammonium (R n NH 4-n + ) cations are often employed as templates for selective cyclization of poly(ethylene glycol) (PEG)-containing substrates into crown ether derivatives [4] , [8] or interlocked molecules (rotaxanes and catenanes) [5] , [6] , [7] , [9] , [10] , typically combined with metathesis reactions. Templates assist not only the selective production of such supramolecular materials [4] , [5] , [6] , [7] , [8] , [9] , [10] but also the precision control of the primary structure of polymers [11] , [12] , [13] , [14] , [15] , [16] , [17] , [18] . For example, we and other groups have recently developed template-assisted precision control of tacticity [15] and monomer sequence [16] , [17] , [18] in conjunction with metal-catalysed living radical polymerization [19] , [20] , [21] , [22] . Cyclopolymerization [23] , [24] , [25] , [26] , [27] , [28] , [29] , [30] , [31] , [32] , [33] , [34] , [35] , [36] is a chain polymerization of bifunctional monomers via alternating propagation process of intramolecular cyclization and intermolecular addition, to give soluble linear polymers consisting of ‘in-chain’ cyclic structures. This strategy affords direct and quantitative incorporation of cyclic units into polymers as repeating units, in sharp contrast to the polymerization of monomers bearing a cyclic pendent group [37] or the postfunctionalization of linear polymers [38] . With the in-chain multiple cyclic units, cyclopolymers potentially show unique functions, for example, polymeric (pseudo-)crown ethers recognize particular cations in a way different from their monomeric counterparts [25] , [32] , [39] . The key for selective vinyl-type cyclopolymerization is to bring the two olefins in a bifunctional monomer to close proximity for effective intramolecular cyclization. This suppresses intermolecular propagation with only one of the two alkene units into pendent olefin-bearing polymers; otherwise the dangling olefin further causes intermolecular crosslinking of polymers to give insoluble gels and/or branched polymers [40] , [41] , [42] , [43] . So far, cyclopolymers with relatively large in-chain rings (at most 20-membered rings) generally required the elaborate design of bifunctional monomers that bring two olefins close, typically through a rigid spacer [29] , [30] , [31] , [32] , except for counterparts with small five- or six-membered rings from 1,6-dienes and 1,6-diynes [33] , [34] , [35] , [36] . Herein, we report cation template-assisted controlled radical cyclopolymerization of poly(ethylene glycol) dimethacrylates (PEG n DMA: CH 2 =C(CH 3 )COO–(CH 2 CH 2 O) n –C(O)C(CH 3 )=CH 2 , n =4–8) as a novel, one-pot and versatile strategy to selectively produce, so-called polymeric pseudo-crown ethers, cyclopolymers with large in-chain PEG rings (each with 19- to 30-membered ether units, 13–100 rings per chain) for efficient and unique cation recognition ( Fig. 1 ). The polymer synthesis is achieved through the specific interaction of the PEG unit with the metal cation. PEGnDMA is treated with metal salts (M + X − ) in polymerization to assume the pseudo-cyclic conformation (PEG n DMA-M + ) via dynamic equilibrium, where the two intramolecular vinyl groups are brought adjacent and are thereby suitably positioned for cycloaddition. The cyclization of PEG n DMA with a template was effective up to 30-membered ‘in-chain’ PEG ring based on eight flexible oxyethyrene units. Typically, ruthenium-catalysed polymerization of K + -template PEG6DMA directly leads to water-soluble linear polymers with narrow molecular weight distributions ( M w / M n ~1.2) and large 24-membered in-chain cyclic PEG units (>97%), without gels or unreacted dangling olefin. The cyclic PEG units efficiently work as nanocavities to interact with alkali metal cations, 1:1 per cyclic unit for Rb + , K + , Na + and Li + or 1:2 for Cs + , and selectively recognize Na + over Li + or Bu 4 N + and K + over Na + under competitive conditions. To our knowledge, this is the first example to apply cation templates for selective and efficient cyclopolymerization of divinyl monomers carrying a long, flexible spacer via the alternating propagation of intramolecular cyclization and intermolecular addition into cyclopolymers containing multiple and large in-chain PEG rings, in sharp contrast to conventional template-directed intramolecular cyclization for crown ether-based supramolecular materials [4] , [5] , [6] , [7] , [8] , [9] , [10] . It should be noted that this template-mediated cyclopolymerization is an efficient, one-pot and selective chemical transformation from common reagents with simple templates to functional cyclopolymers. 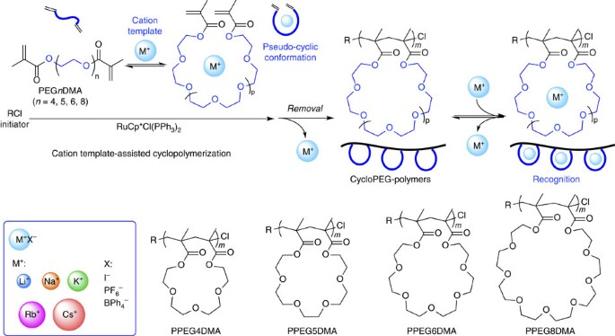Figure 1: Cation template-assisted cyclopolymerization for polymeric pseudo-crown ethers. PEGnDMA efficiently interacts with metal cations toin situform pseudo-cyclic conformation with the adjacent location of the two olefins, which induces the alternating propagation process of intramolecular cyclization and intermolecular addition to selectively give linear polymers comprising large in-chain cyclic PEG rings (up to 30 membered). Thus, cyclic PEG polymers behave as polymeric pseudo-crown ethers to perform unique cation recognition dependent on the ring size. Figure 1: Cation template-assisted cyclopolymerization for polymeric pseudo-crown ethers. PEG n DMA efficiently interacts with metal cations to in situ form pseudo-cyclic conformation with the adjacent location of the two olefins, which induces the alternating propagation process of intramolecular cyclization and intermolecular addition to selectively give linear polymers comprising large in-chain cyclic PEG rings (up to 30 membered). Thus, cyclic PEG polymers behave as polymeric pseudo-crown ethers to perform unique cation recognition dependent on the ring size. Full size image Cation template monomers PEG n DMAs, dimethacrylates carrying a PEG spacer unit [–(CH 2 CH 2 O) n –] of a well-defined degree of polymerization ( n =4, 5, 6, 8) were employed as monomers for cation template-assisted cyclopolymerization. The interaction between PEG n DMA and metal cations was first evaluated ( Fig. 2 , Supplementary Fig. S1–S3 and Supplementary Table S1 ). In general, 18-crown-6, a cyclic crown ether consisting of six ethylene oxide units, efficiently recognizes potassium cation (K + ) because the inner pore is best fit in size for K + (ref. 4 ). PEG6DMA was thus mixed with KPF 6 in acetone- d 6 /cyclohexanone (1/1, v/v) to analyse its interaction with K + by proton nuclear magnetic resonance spectroscopy ( 1 H NMR) ( Fig. 2a,b ). The protons ( c , d′ , and d ) assignable to the PEG segment shifted to downfield by +0.04 p.p.m., larger than the accompanying shift in the chain-end methacrylate groups ( a , b : <~0.01 p.p.m. ), suggesting that the PEG spacer efficiently interacts with K + . The stoichiometry of the interaction was 1:1 (one cation per PEG6DMA ), as determined by Job’s method based on the chemical shift change of the PEG proton (peak c ) and the molar fraction of PEG units ( χ ): [ PEG6DMA ]/[KPF 6 ]=10/0–10/1, [ PEG6DMA ]+[KPF 6 ]=10 mM ( Fig. 2c ); the plot showed a maximum at χ =0.5. The association constant ( K a ) was estimated as ~70 M −1 by 1 H NMR titration experiment of PEG6DMA with K + ( Supplementary Figs S2 and S3 and Supplementary Table S1 ). Similarly, PEG5DMA and PEG8DMA also captured K + via 1:1 interaction, whereas PEG4DMA was totally ineffective ( Fig. 2c ), suggesting that K + was suited for PEG n DMAs carrying 5–8 ethylene oxide units. In addition, PEG6DMA recognized K + more efficiently than Na + and Li + (NaI: K a =~30 M −1 ; LiI: no specific interaction, Supplementary Table S1 ). 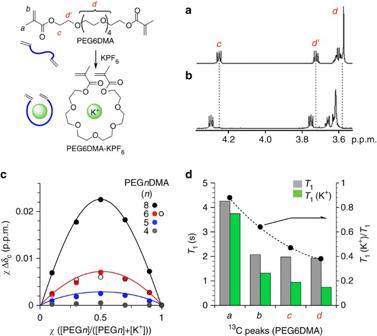Figure 2: Interaction of PEGnDMA with a K+template. 1H NMR spectra ofPEG6DMA(a) andPEG6DMAwith KPF6(b) in acetone-d6/cyclohexanone (1/1, v/v) at 30 °C. The proton signals of the ethylene oxide unit onPEG6DMAshifted to downfield in the presence of KPF6. (c) Job plots were obtained from1H NMR measurements of PEGnDMAs with KI (filled circle:n=4 (grey), 5 (blue), 6 (red), 8 (black)) or KPF6(n=6: open black circle) ([PEGnDMA]0+[K+]0=10 mM). PEGnDMAs efficiently interact with K+ via 1:1 per PEG unit, except for PEG4DMA. (d) Longitudinal relaxation time (T1) measurements of the carbons forPEG6DMA(grey bar) andPEG6DMAwith KPF6(green bar) by13C NMR.T1(K+)s forPEG6DMAwith KPF6turned smaller than those forPEG6DMAalone, meaning the decreasing mobility ofPEG6DMAwith K+. Importantly, efficient interaction of the PEG segment (peaks:c,d) with K+was supported by the ratio (T1(K+)/T1: filled circle) for the PEG smaller than that for methacrylates (peaks:a,b). Figure 2: Interaction of PEGnDMA with a K + template. 1 H NMR spectra of PEG6DMA ( a ) and PEG6DMA with KPF 6 ( b ) in acetone- d 6 /cyclohexanone (1/1, v/v) at 30 °C. The proton signals of the ethylene oxide unit on PEG6DMA shifted to downfield in the presence of KPF 6 . ( c ) Job plots were obtained from 1 H NMR measurements of PEG n DMAs with KI (filled circle: n =4 (grey), 5 (blue), 6 (red), 8 (black)) or KPF 6 ( n =6: open black circle) ([PEGnDMA] 0 +[K + ] 0 =10 mM). PEG n DMAs efficiently interact with K+ via 1:1 per PEG unit, except for PEG4DMA. ( d ) Longitudinal relaxation time ( T 1 ) measurements of the carbons for PEG6DMA (grey bar) and PEG6DMA with KPF 6 (green bar) by 13 C NMR. T 1 (K + )s for PEG6DMA with KPF 6 turned smaller than those for PEG6DMA alone, meaning the decreasing mobility of PEG6DMA with K + . Importantly, efficient interaction of the PEG segment (peaks: c , d ) with K + was supported by the ratio ( T 1 (K + )/ T 1 : filled circle) for the PEG smaller than that for methacrylates (peaks: a , b ). Full size image The local mobility of PEG6DMA was further evaluated with longitudinal relaxation time ( T 1 ) of the carbons ( a – d ) in the presence of KPF 6 by 13 C NMR ([ PEG6DMA ]/[KPF 6 ]=1/2; Fig. 2d , Supplementary Fig. S4 and Supplementary Table S2 ). For all the carbons, T 1 s with K + [ T 1 (K + )s] were smaller than those without K + ( T 1 s). As plotted in Fig. 2d , the ratio [ T 1 (K + )/ T 1 s] for PEG units ( c and d ) was much smaller than that for methacrylate moieties ( a and b ), demonstrating that the PEG segment predominantly binds K + . The same conclusion was also supported by ultraviolet–visible analysis ( Supplementary Fig. S5 ). Template-assisted cyclopolymerization Cation template-assisted cyclopolymerization of PEG6DMA was carried out in conjunction with a ruthenium catalytic system [RuCp*Cl(PPh 3 ) 2 / n -Bu 3 N] and a chloride initiator [H-(MMA) 2 -Cl] [44] in cyclohexanone at 40 °C. Following the cation recognition data, the bifunctional monomer was mixed with K + at 1/1 molar ratio in cyclohexanone to in situ transform a pseudo-cyclic monomer with K + template. Without further isolation of the complex, the mixture was directly polymerized under dilute conditions ([ PEG6DMA ] 0 =25–100 mM) ( Fig. 3 , Table 1 and Supplementary Fig. S6 ). The targeted degree of polymerization ( DP =[ PEG6DMA ] 0 /[H-(MMA) 2 -Cl] 0 ) was set at 12.5–100, that is, the number of ‘in-chain’ cyclic units per polymer=12.5, 25, 50 and 100. The polymerization proceeded smoothly and homogeneously in high yield (~90% conversion in 30–56 h) without any gelation, independent of the targeted DP . The number-average molecular weight of products increased with increasing conversion and was proportional to the targeted DP s ( M n =7,500–31,100; M w / M n =1.1–1.5; by size-exclusion chromatography (SEC); Fig. 3a ). Thus, this ruthenium-mediated cyclopolymerization with metal cation templates was efficiently controlled to lead to linear polymers. Such a fine control was also maintained with excess cation over the monomer ([ PEG6DMA ] 0 /[KPF 6 ] 0 =1/1, 1/2, 1/5; DP =12.5; M w / M n =<1.2). In contrast, direct polymerization of PEG6DMA in a cation-free system (entries 1,7) was retarded and resulted in high-molecular weight products with bimodal distribution ( M w / M n : ~2.0) and/or some gels, suggesting intermolecular crosslinking of linear chains. 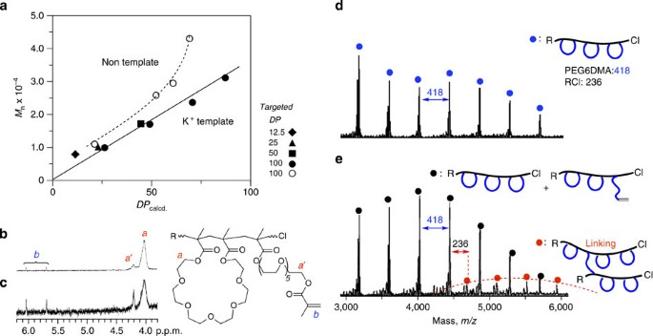Figure 3: K+template-assisted cyclopolymerization ofPEG6DMA. (a) Number-averaged molecular weight as a function of calculated degree of polymerization (DPcalcd.): [PEG6DMA]/[KPF6]/[H-(MMA)2-Cl (RCl)]/[RuCp*Cl(PPh3)2]/[n-Bu3N]=25–100/0–100/2.0, 1.0/0.5/20 mM in cyclohexanone at 40 °C.1H NMR (b,c) and MALDI-TOF-MS (d,e) spectra of initial PPEG6DMA samples (TargetedDP=13) obtained with a KPF6template (b,d) and without the template (c,e). The K+template-assisted polymerization ofPEG6DMAsmoothly and selectively gave linear PPEG6DMA with high cyclization efficiency (>97%, (d): filled blue circle), whereas the direct polymerization ofPEG6DMAinduced intermolecular linking reaction of polymer chains to lead to high-molecular weight products including dangling olefins (~20%, (e): filled black and red circles). Figure 3: K + template-assisted cyclopolymerization of PEG6DMA . ( a ) Number-averaged molecular weight as a function of calculated degree of polymerization ( DP calcd. ): [ PEG6DMA ]/[KPF 6 ]/[H-(MMA) 2 -Cl (RCl)]/[RuCp*Cl(PPh 3 ) 2 ]/[ n -Bu 3 N]=25–100/0–100/2.0, 1.0/0.5/20 mM in cyclohexanone at 40 °C. 1 H NMR ( b , c ) and MALDI-TOF-MS ( d , e ) spectra of initial PPEG6DMA samples (Targeted DP =13) obtained with a KPF 6 template ( b , d ) and without the template ( c , e ). The K + template-assisted polymerization of PEG6DMA smoothly and selectively gave linear PPEG6DMA with high cyclization efficiency (>97%, ( d ): filled blue circle), whereas the direct polymerization of PEG6DMA induced intermolecular linking reaction of polymer chains to lead to high-molecular weight products including dangling olefins (~20%, ( e ): filled black and red circles). Full size image Table 1 K + template-assisted cyclopolymerization of PEG n DMA. Full size table Microscopic structures of products were analysed by matrix-assisted laser desorption ionization time-of-flight mass spectrometry (MALDI-TOF-MS) and 1 H NMR spectroscopy, to determine the intramolecular cyclization efficiency (CE) [18] . Figure 3d shows a typical MALDI spectrum of poly( PEG6DMA ) obtained with K + at the initial stage (targeted DP =12.5; ~30% conversion in entry 2). The sample exhibited a single series of peaks (blue filled circle), regularly separated by the molar mass of the monomer (418.5). The absolute mass of each peak was equal to that expected for the PEG6DMA polymer capped with one initiator fragment [H–(MMA) 2 –] at the α-end and one chlorine at the ω-end ( cf . m / e for H–(MMA) 2 –+Cl: 236.7), plus a sodium ion from externally added salt for ionization. The products showed 1 H NMR signals of the methacrylate backbone (CH 3 -: 0.7–1.2 p.p.m. ; -CH 2 -: 1.4–2.0 p.p.m.) and the cyclized PEG units (-CH 2 CH 2 O-: 3.4–3.7 p.p.m. ; -COOC H 2 CH 2 O- ( a + a′ : 4.0–4.2 p.p.m.) but virtually without olefin signals ( b : 5.7, 6.0 p.p.m.) ( Fig. 3b and Supplementary Fig. S7 ). From the signal intensity ratio b /( a + a′ ), the dangling (unreacted) olefin content was estimated as 4.9% for an initial sample (conversion ~30%, Fig. 3b ) and 2.4% for a final sample (conversion 87%, Supplementary Fig. S7 ). The decrease with conversion suggests that the observed olefin might be located at the ω -terminal unit, where one methacrylate in the monomer is consumed by intermolecular propagation, whereas another stands by for intramolecular cyclization. These results indicate that at high CE (>97%), that is, nearly without intermolecular crosslinking, almost all methacrylate units of PEG6DMA are cyclopolymerized into linear cyclopolymers with a large 24-membered ‘in-chain’ cyclic PEG unit. Separate experiments also showed that CE was as high as 95–99%, invariably independent of the template feed ([ PEG6DMA ] 0 /[KPF 6 ] 0 =1/1–1/5) and targeted DP ([ PEG6DMA ] 0 /[initiator] 0 =12.5–100). On the contrary, samples prepared without K + showed two series of mass peaks from the initial stage of the polymerization (~30% conversion in entry 1; Fig. 3e ). In addition to a series of cyclopoly( PEG6DMA ) with one α -end initiator fragment (black filled circles), another series in the higher-molecular-weight region (red filled circles) was consistent with polymers carrying two initiator fragments indicative of intermolecular crosslinking (coupling) of two chains. These samples showed large 1 H NMR signals of dangling olefins ( b ) and adjacent methylene units ( a′ ) ( Fig. 3c ), in which, without cation template, ~20% monomer units were not intramolecularly cyclized even under diluted monomer conditions (25 mM). We further examined cyclopolymerization with other templates (LiPF 6 , NaPF 6 and CsBPh 4 ) and/or PEG dimethacrylate monomers of different spacer length (PEG n DMA; n =4, 5, 8) ( Table 1 , Supplementary Table S3 and Supplementary Fig. S8 ). For PEG6DMA , KPF 6 (K + ) was the most effective template; CE: 85% (LiPF 6 ), 93% (NaPF 6 ), 95% (KPF 6 ), 85% (CsBPh 4 );<80% (no template). Random and block copolymerizations with methyl methacrylate (MMA) were also possible (random: MMA/ PEG6DMA =25/13 or 75/13; M w / M n =1.2; block (from MMA): MMA/ PEG6DMA =100/13; M w / M n =1.3) ( Supplementary Figs S9 and S10 ). The K + template was also applicable to PEG5DMA and PEG8DMA to give linear cyclopolymers carrying 21- and 30-membered in-chain PEG rings, respectively ( cf . 24-membered rings with PEG6DMA ). In contrast, the cyclopolymerization of PEG4DMA occurred in fairly high CE independent of templates (even without a template cation), because the restricted conformation from the relatively short spacer renders the two vinyl groups intramolecularly close to each other without the assistance of a template [28] , [43] . The template effect on the conformation of PEG n DMA/K + pairs was confirmed in dynamics calculation (software: Schrödinger MacroModel 9.5; duration 10 6 fs; 300 K) ( Supplementary Figs S11 and S12 ). For example, the inter-olefin distance in PEG6DMA in the presence of K + was in the range of 3.0–7.0 Å (>99% probability) and 4.7 Å ( d avg ) on average, whereas without K + the distance fluctuated more widely from 3.0 to 10 Å or beyond (>10 Å in ~50% probability; d avg =8.7 Å). Similar simulation results were obtained for PEG5DMA and PEG8DMA . Additionally, d avg for PEG6DMA decreased as a function of cations: template free (8.7 Å)>Cs + (7.9 Å)>Na + (5.2 Å)>K + (4.7 Å). Note that the CE in cyclopolymerization increased in the opposite order, demonstrating that the shorter d avg is the more favored cyclopropagation. Properties Owing to some steric requirement on cyclopropagation and/or the resulting cyclic repeat units, PPEG n DMAs exhibited stereoregularity different from that of the linear pendant counterparts (PPEG n MA) [18] . Analysed by 1 H and 13 C NMR ( Table 1 , Supplementary Fig. S7 ), PPEG n DMAs ( n =5, 6, 8) were more heterotactic than PPEG n MA ( n = 4 , 8.5 ) ( mm / mr / rr =2.2/35.6/62.2 ( PEG5DMA ), 2.5/41.0/56.4 ( PEG6DMA ), 2.9/36.6/60.5 ( PEG8DMA ), 2.1/30.9/67.0 (PEG 4 MA), 1.9/29.9/68.2 (PEG 8.5 MA)). Although the stereoregularity for PPEG n MA was independent of the pendant length, that for PPEG n DMAs was dependent on the ring size ( n ). Cyclopolymerization expectedly reduced the thermal mobility of the spacer PEG units. Determined by 13 C NMR, spin-lattice relaxation time ( T 1 ) of the PEG spacer carbons in PPEG6DMA was 0.51 s, much shorter than those for the monomer (1.93 s) and for the linear pendants in PPEG 8.5 MA (1.68 s) ( Supplementary Table S4 ). Within the cyclopolymers PPEGnDMA, T 1 decreased with decreasing number of oxyethylene units ( n ): T 1 ( n )=0.48 (5), 0.51 (6), 0.68 (8); the shorter the spacer (the smaller ring size), the more limited the thermal mobility. The lowered mobility also supports the formation of cyclopolymers with ‘in-chain’ polyether rings. Because of the hydrophilic and thermosensitive PEG units, cyclopolymers of PEG6DMA and PEG8DMA were soluble in water at room temperature (r.t.) but underwent reversible, hysteresis-free phase transition in a narrow temperature range where the lower critical solution temperature (LCST) was 35 and 50 °C, respectively ( Supplementary Fig. S13 ). The LCST for PPEG6DMA was between those for non-cyclic counterparts from PEG2MA (~26 °C) and PEG3MA (~52 °C) [45] , [46] . PPEG6DMA might provide attractive thermosensitive amphiphilic biomaterials with LCST close to the human body temperature. Ion recognition Given their consecutively placed in-chain crown ether units, recognition of metal cations was examined for PPEGnDMAs obtained with the K + template ( Fig. 4 , Supplementary Figs S14–S18 and Supplementary Table S5 ). Thus, interaction of PPEG6DMA ( DP =12.5; M n =7,900) with alkali metal salts (LiI, NaI, KI, KPF 6 and RbI; separately mixed with the polymer) was followed by 1 H NMR spectroscopy in an acetone- d 6 /cyclohexanone mixed solvents (1/1, v/v) at 30 °C ( Fig. 4a ). Exposure to their cations induced downfield shifts in the PEG protons, indicative of cation encapsulation into the cyclic backbone cavity. The symmetrical Job plots peaked at χ =0.5 (molar fraction of the ring unit) demonstrated a 1:1 stoichiometeric interaction between a cation guest and an in-chain ring host. The cyclopolymer exhibited a stronger cation affinity than its monomer, judged from the association constant by 1 H NMR ( K a (M −1 ): ~130 versus ~70 with KPF 6 ; ~30 versus ~0 (no interaction) with LiI). Equally important, K + fitted to the cyclopolymer more efficiently than Li + ( K a (M −1 ): ~130 (K + ) versus ~30 (Li + )) owing to the ring size suitable for K + . The 1:1 cation binding also occurred in an MMA/ PEG6DMA random copolymer (75/13 ratio in DP ) consisting of the same cycloPEG units and the K a (~140 M −1 ) was similar to that with a PEG6DMA homopolymer. This indicates that each in-chain ring captures K + independently without interfering effects with the neighbouring units. The thermal mobility ( T 1 ) of cycloPEG units decreased on K + recognition ( Supplementary Table S4 ). 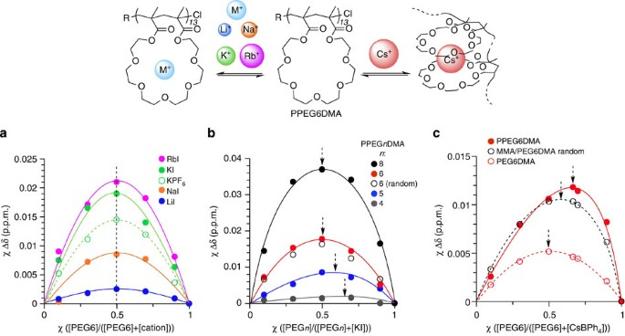Figure 4: Cation recognition with PPEGnDMA. Job plots were obtained from1H NMR measurements of PPEGnDMA (n=4–8) with metal cations in acetone-d6/cyclohexanone (1/1) at 30 °C ([cyclic PEG units on PPEGDMA]0+[cation]0=10 mM). (a) Job plots for PPEG6DMA with various metal cations (LiI, NaI, KPF6, KI, RbI) support 1:1 recognition of their cations per cycloPEG unit. (b) Effects of spacer length (n) of PPEGnDMA (homopolymer: filled circles; a MMA/PEG6DMA(75/13) random copolymer: open circle) on KI recognition (dash arrow: peak top). (c) CsBPh4recognition with PPEG6DMA (filled red circle), a MMA/PEG6DMA(75/13) random copolymer (open black circle),PEG6DMA(open red circle) (dash arrow: peak top). PPEGnDMA efficiently recognized a Cs+per two neighbouring cyclic PEG units due to the local high density. Figure 4: Cation recognition with PPEGnDMA. Job plots were obtained from 1 H NMR measurements of PPEG n DMA ( n =4–8) with metal cations in acetone- d 6 /cyclohexanone (1/1) at 30 °C ([cyclic PEG units on PPEGDMA] 0 +[cation] 0 =10 mM). ( a ) Job plots for PPEG6DMA with various metal cations (LiI, NaI, KPF 6 , KI, RbI) support 1:1 recognition of their cations per cycloPEG unit. ( b ) Effects of spacer length ( n ) of PPEG n DMA (homopolymer: filled circles; a MMA/ PEG6DMA (75/13) random copolymer: open circle) on KI recognition (dash arrow: peak top). ( c ) CsBPh 4 recognition with PPEG6DMA (filled red circle), a MMA/ PEG6DMA (75/13) random copolymer (open black circle), PEG6DMA (open red circle) (dash arrow: peak top). PPEG n DMA efficiently recognized a Cs + per two neighbouring cyclic PEG units due to the local high density. Full size image However, the K + recognition by PPEGnDMA was dependent on the ring size ( n ) ( Fig. 4b ). The stoichiometry (K + :cycloPEG unit) changed from 1:1 to 1:2 as n decreased from 6 to 4, judged from the fact that the Job-plot maximum shifted from χ =0.5 to 0.66. PPEG8DMA with larger in-chain rings captured K + in 1:1 stoichiometry four times more efficiently than PPEG6DMA ( K a (M −1 )=~460 (PPEG8DMA), ~130 (PPEG6DMA)), though the 30-membered ring from PEG8DMA seemed too large for K + at first glance. Uniquely, the binding with PPEG8DMA preferentially occurred via the middle oxyethylene units ( d : -(C H 2 C H 2 O) n -) rather than via those adjacent to the ester linkages ( c : -COOC H 2 CH 2 O-), as the K a for d is larger than the K a for c ( K a (M −1 )=~110 ( c ) versus ~460 ( d )). This is because the 30-membered ring is spacious and flexible enough to mobilize some of the middle ether units, assuming a conformation better fit for the cation. In contrast, PPEG6DMA with rigid 24-membered rings apparently needs all the ring units (both middle ( d ) and ester-bound ( c )) to capture K + , as indicated by virtually no difference among their binding constants. The association constant of PPEGnDMA to K + (maximum: K a (M −1 )=~460) was smaller than that of crown ether derivatives with similar ring size under identical conditions (that is, dibenzo-21-crown-7-ether to K + : K a (M −1 )=~2.0 × 10 4 ) probably owing to strained conformation of the in-chain cyclized PEG units. Recognition of a caesium cation (CsBPh 4 ) was further examined with cycloPEG homopolymers (PPEG6DMA, PPEG8DMA), an MMA/ PEG6DMA (75/13) random copolymer and their monomers ( Fig. 4c , Supplementary Fig. S18 ). Their homopolymers bound one Cs + with two cycloPEG units (peak maximum in Job plots: χ =0.66), whereas their monomers did Cs + via 1:1 stoichiometry (Cs + : cycloPEG) as well as the other cations (Na + , K + , Rb + ; Supplementary Fig. S1 ). Such specific 1:2 recognition (Cs + :cycloPEG) was independent of counter anion and solvents (CsI: recognized with two cycloPEG in CD 3 OD). In contrast, the random copolymer competitively involved both 1:1 recognition and 1:2 counterpart (Cs + :cycloPEG), where the peak maximum of the Job plot was at ~0.6 between 0.66 and 0.5. 18-Crown-6 in turn selectively showed 1:1 recognition. Thus, the unique 1:2 recognition for Cs + is attributed to the local high concentration of cycloPEG units per chain. Confirmed by dynamic light scattering, PPEG6DMA in the presence of K + or Cs + had hydrodynamic radius ( R h ) almost identical to PPEG6DMA alone ( R h =6.3 nm (K + or Cs + ), 7.9 nm (non cation) in acetone), indicating that cycloPEG polymers intramolecularly grasped Cs + with the two neighbouring cycloPEG units within a single chain. Selective and competitive ion recognition The efficiency and selectivity in the cation recognition by PPEG6DMA was further evaluated in competitive recognition. Thus, in cyclohexanone/acetone- d 6 (1/1, v/v), the polymer was mixed with an equimolar mixture of Na and another alkali metal cation, and the selectivity was evaluated in monitoring the sodium guest by 23 Na NMR spectroscopy ( Fig. 5 ); obviously, 1 H or 13 C NMR is totally useless in this analysis, because there was little difference in the chemical shift between cyclic PEG units with Na and with another cation. This method will also provide evidence for recognition not from the host (PEG by NMR) but from the guest (cation). 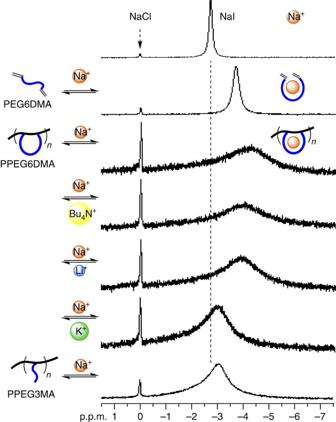Figure 5: Competitive cation recognition with PPEG6DMA. 23Na NMR measurements of NaI with PPEG6DMA in the presence of other cations (Bu4NI, LiI, KI) were conducted in acetone-d6/cyclohexanone (1/1, v/v) at 30 °C. Owing to the ‘in-chain’ cyclic PEG structure, PPEG6DMA recognized NaI more efficiently thanPEG6DMA(monomer) and poly(triethylene glycol methyl ether methacrylate) (PPEG3MA: linear pendant). Additionally, PPEG6DMA performed Na+recognition selective over Bu4N+or Li+, and K+recognition over Na+. Figure 5: Competitive cation recognition with PPEG6DMA. 23 Na NMR measurements of NaI with PPEG6DMA in the presence of other cations (Bu 4 NI, LiI, KI) were conducted in acetone- d 6 /cyclohexanone (1/1, v/v) at 30 °C. Owing to the ‘in-chain’ cyclic PEG structure, PPEG6DMA recognized NaI more efficiently than PEG6DMA (monomer) and poly(triethylene glycol methyl ether methacrylate) (PPEG3MA: linear pendant). Additionally, PPEG6DMA performed Na + recognition selective over Bu 4 N + or Li + , and K + recognition over Na + . Full size image In the presence of PPEG6DMA, the Na signal of NaI shifted upfield by Δδ=–1.53 p.p.m. and broadened (half width: 350 Hz from 19.8 Hz (polymer-free salt)). The peak shift and broadening was larger than those with the monomer (–0.96 p.p.m. and 40 Hz) and with PPEG3MA (a linear pendant counterpart to PPEG6DMA: –0.34 p.p.m. and 135 Hz), again demonstrating the efficient cation binding by 23 Na NMR. More importantly, PPEG6DMA selectively recognized Na + over Li + or Bu 4 N + and in turn did K + over Na + in competitive experiments where an equimolar mixture of the probe and another cation was exposed to the cyclopolymer. The upfield shift and broadening for the sodium signal of NaI with PPEG6DMA were still maintained in the presence of Bu 4 NI and LiI. However, KI made the sodium signal shifting to downfield (close to original position) again and narrow. This implies that the presence of competing cations does not seriously interfere with the recognition of a preferred cation and that the cation selectivity in PPEG6DMA increases in the order Bu 4 N<Li<Na<K. In addition, the in-chain cyclic PEG units are essential for the selective recognition, as PPEG3MA turned out poorly selective in cation recognition ( Supplementary Fig. S19 ). Cyclopolymerization of divinyl monomers for linear polymers containing in-chain cyclic structures essentially undergoes an alternating propagation process of intramolecular cyclization and intermolecular addition, in which the efficient intramolecular cyclization is a key step to prevent the intermolecular crosslinking of polymer chains. In cation template-assisted cyclopolymerization, a potassium cation (K + ) effectively interacts with PEG-bearing dimethacrylates, PEG n DMA ( n =5–8) to transform the random conformation into the pseudo-cyclized counterpart. As a result, the two vinyl groups come close to be suitable for intramolecular cyclization, which is also supported by molecular dynamics calculation. Owing to high tolerance to polar functional groups including metal cations [19] , [20] , a ruthenium catalytic system efficiently induces controlled radical cyclopolymerization of PEG n DMA in the presence of a potassium cation to directly give linear polymers (PPEG n DMA) bearing large (19–30 membered) in-chain cyclic PEG rings with controlled molecular weight. The resulting PPEG n DMAs further work as unique nanocavities to recognize metal cations, more efficiently and selectively than their linear pendant counterparts and an original monomer. In the present design, the binding constant to metal cations is smaller than that with corresponding crown ethers. This is probably because cyclized PEG rings in PPEG n DMAs have steric strain and/or irregular conformation originating from the ill-controlled stereoregularity, though PPEG n DMAs ( n =5–8) obtained with a potassium template are more heterotactic than linear counterparts (PPEGMAs). Thus, development of stereoregular cyclopolymerization of PEG n DMA would be important for resolving that issue; such a polymerization system could produce cycloPEG polymers with highly regulated ring conformation to induce cooperative recognition of cationic compounds more efficiently and selectively compared with conventional crown ethers. In addition, cation template-assisted polymerization is quite versatile to afford various primary structures from simple cyclopolymers to random and block copolymers containing cyclized PEG n DMA units. In the future, cycloPEG-bearing microgel star polymers might be useful as efficient and selective scavengers to extract (or remove) metal cations from solution, because microgel star polymers potentially behave as nanocapsules to capture molecules and can be easily recovered from solution by modulating the arm species [41] . In conclusion, we have successfully developed cation template-mediated, controlled radical cyclopolymerization of PEG spacer-bearing dimethacrylates, PEG n DMA ( n =4–8), for polymeric pseudo-crown ethers performing unique cation recognition. The synergistic marriage of supramolecular chemistry and polymer chemistry opens a new efficient strategy to create well-defined functional cyclopolymers from common reagents with simple template molecules. Multi-control of primary structures and/or tailor-made design of three-dimensional architectures would further advance cycloPEG-based polymers as novel functional macromolecules to innovate on molecular recognition. Materials Triethylene glycol monomethyl ether (Aldrich, purity >95%), tetraethylene glycol (TCI, purity >95%), pentaethylene glycol (TCI, purity >95%), hexaethylene glycol (Aldrich, purity >97%), octaethylene glycol (Wako, purity >97%), tetrahydrofuran (Wako; dehydrated), diethyl ether (Wako, purity >99.5%), sodium sulphate (Wako, purity >99%) and 25% ammonia solution (Wako) were used as received. Methacryloyl chloride (TCI, purity >80%) and triethylamine (TCI, purity >99%) were purified by distillation before use. MMA (TCI; purity >99%) was dried overnight over calcium chloride and purified by double distillation under reduced pressure from calcium hydride before use. Poly(ethylene glycol) dimethacrylate (PEG n DMA: n =[-(CH 2 CH 2 O)-]/[PEGnDMA]=4, 5, 6, 8) was synthesized as shown below. Triethylene glycol methyl ether methacrylate (PEG3MA) was prepared according to the literature [45] . Poly(ethylene glycol) methyl ether methacrylate (PEG n MA: M n =475 ( n = 8.5 ); M n =300 ( n = 4 ); Aldrich) was purified by an inhibitor remover column (product no. : 311332, Aldrich) and was degassed by vacuum-argon purge cycles before use. Ethyl α-chlorophenylacetate (ECPA: Aldrich; purity >97%) was purified by distillation under reduced pressure before use. H-(MMA) 2 -Cl was prepared according to the literature [44] . RuCp*Cl(PPh 3 ) 2 (Cp*: pentamethylcyclopentadienyl, Aldrich, purity >97%) was used as received and was handled in a grove box under a moisture- and oxygen-free argon atmosphere (H 2 O<1 p.p.m., O 2 <1 p.p.m.). n -Bu 3 N (TCI, purity>98%) was degassed by vacuum-argon purge cycles before use. Tetralin (1,2,3,4-tetrahydronaphthalene) (Kisida Chemical, purity >98%), as an internal standard to check the conversion of PEGn(D)MA by 1 H NMR, was dried over calcium chloride overnight and distilled twice from calcium hydride. Cyclohexanone (Wako, purity >99%) was dried on molecular sieves 4A (Wako) and degassed by vacuum-argon purge cycles before use. Methanol (Wako, purity>99.8%) and regenerated cellulose dialysis membranes (Spectra/Por 7; molecular weight cut off (MWCO) 1,000) for polymer purification were used as received. Lithium iodide (LiI: Aldrich; purity >99%), sodium iodide (NaI: Aldrich; purity >99.9%), potassium iodide (KI: Wako; purity >99%), potassium hexafluorophosphate (KPF 6 : Aldrich; purity >98%), rubidium iodide (RbI: Aldrich; purity >99.9%), caesium iodide (CsI: Aldrich; purity >99.9%), caesium tetraphenylborate (CsBPh 4 : Aldrich; purity >98%), 18-crown-6 (Wako, purity >98%), dibenzo-21-crown-7-ether (TCI, purity >96%) and acetone- d 6 (CIL) were used as received. Monomer synthesis A typical procedure for PEG6DMA was given: in a 200-ml round-bottomed flask filled with argon, methacryloyl chloride (94.6 mmol, 9.1 ml) was added dropwise to a solution of hexaethylene glycol (31.5 mmol, 10 ml) and triethylamine (94.6 mmol, 6.3 ml) in dry tetrahydrofuran (70 ml) at 0 °C. The reaction mixture was stirred at 0 °C for 2 h and at 25 °C for an additional 22 h, and then evaporated under reduced pressure. The concentrated crude was diluted with diethyl ether (150 ml) and washed with water (150 ml). The aqueous layer was separated and further extracted with diethyl ether (150 ml). The combined ether solution was washed with 200 ml of 25% ammonia water three times and with 200 ml of distilled water once, and was dried on sodium sulphate overnight. Into the purified ether solution of PEG6DMA , dried cyclohexanone was added. The solution was then evaporated under reduced pressure to remove the ether to give cyclohexanone solution of PEG6DMA for cyclopolymerization. 1 H NMR (500 MHz, acetone- d 6 , r.t., δ =2.05 p.p.m. (acetone)): δ 6.08 (m, olefin, 2H), 5.62 (m, olefin, 2H), 4.24 (t, J =4.8 Hz, 4H, -COOCH 2 CH 2 O-), 3.71 (t, J =4.8 Hz, 4H, -COOCH 2 CH 2 O-), 3.62–3.56 (m, 16H, -OCH 2 CH 2 O-), 1.92 (m, 6H, -CCH 3 ). 13 C NMR (125 MHz, acetone- d 6 , r.t., δ =206.5 p.p.m. (acetone)): δ 168.0, 138.0, 126.3, 72.0, 70.3, 65.3, 19.2. Electrospray ionization mass spectrometry m / z ([M+Na] + ): calcd. for C 20 H 34 O 9 Na 441.2, found 441.2. See Supplementary Methods for synthesis and characterization of other monomers. Polymerization Cation template-assisted living radical cyclopolymerization of PEGnDMA ( n =4–8) was carried out by the syringe technique under argon in baked glass tubes equipped with a three-way stopcock. PEG n DMA was pre-mixed with KPF 6 in cyclohexanone at a predetermined ratio ([PEG n DMA]/[KPF 6 ]=1/1–1/5) to give a cyclohexanone solution of PEG6DMA interacting with KPF 6 . A typical procedure for PPEG6DMA ( DP =12.5) was given: RuCp*Cl(PPh 3 ) 2 (0.005 mmol, 4.0 mg) was placed in a 30-ml glass tube. Into the tube, cyclohexanone (8.7 ml), tetralin (0.1 ml), a 400-mM toluene solution of n -Bu 3 N (0.2 mmol, 0.5 ml), a 789 mM cyclohexanone solution of PEG6DMA with KPF 6 ([ PEG6DMA ]=0.25 mmol, [KPF 6 ]=0.5 mmol, 0.32 ml), and a 57.6 mM toluene solution of H-(MMA) 2 -Cl (0.02 mmol, 0.35 ml) were added sequentially in this order at 25 °C under argon. The tube containing the mixture (total volume: 10 ml) was placed in an oil bath at 40 °C. In predetermined intervals, a small portion of the reaction mixture was sampled and cooled to −78 °C to terminate the reaction. The conversion of PEG6DMA was then determined by 1 H NMR measurement with an internal standard (tetralin) in CDCl 3 at r.t. After 56 h (conversion=87%), the quenched reaction mixture was evaporated to dryness under reduced pressure. The resulting crude was first fractionated by preparative SEC in N,N′-dimethylformamide (DMF) and then dialysed in water with a regenerated cellulose membrane (Spectra/Por 7; MWCO 1,000) for 5 days. The inner solution was evaporated to dryness under reduced pressure to give PPEG6DMA. SEC (DMF, 0.01 M LiBr): M n =7900, g mol −1 ; M w / M n =1.20. 1 H NMR [500 MHz, CDCl 3 , δ =7.26 (CHCl 3 )]: δ 6.2, 5.6 (olefin), 4.2–4.0 (-COOCH 2 CH 2 O-), 3.8–3.5 (-OCH 2 CH 2 O-), 2.1–1.3 (-CH 2 CCH 3 ), 1.3–0.8 (-CCH 3 ). CE=~99%. 13 C NMR [125 MHz, CDCl 3 , δ =77.0 (CHCl 3 )]: δ 178.2–175.5 (C=O), 71.1-70.2 (-OCH 2 CH 2 O-), 68.8–68.4 (-COOCH 2 CH 2 O-), 64.6–63.8 (-COOCH 2 CH 2 O-), 55.5–52.0 (-CH 2 C(CH 3 )CO-), 45.6–44.5 (-CH 2 C(CH 3 )CO-), 22.6–16.0 (-CH 3 ). mm / mr / rr =2.5/41.0/56.4. See Supplementary Methods for the synthesis and characterization of other polymers. Characterization The molecular weight distribution, M n and M w / M n ratios of polymers were measured by SEC in DMF containing 10 mM LiBr at 40 °C (flow rate: 1 ml min −1 ) on three linear-type polystyrene gel columns (Shodex KF-805L; exclusion limit=4 × 10 6 ; particle size=10 μm; pore size=5,000 Å; 0.8 cm i.d. × 30 cm) that were connected to a Jasco PU-2080 precision pump, a Jasco RI-2031 refractive index detector and a Jasco UV-2075 ultraviolet/visible detector set at 270 nm. The columns were calibrated against ten standard poly(MMA) samples (Polymer Laboratories; M n =1,000–12,00,000; M w / M n =1.06–1.22). Polymer samples to analyse the structure and investigate the cation recognition were fractionated by preparative SEC (column: Shodex K-2003; exclusion limit=7 × 10 4 ; particle size=6 μm; pore size=500 Å; 2.0 cm i.d. × 30 cm, eluent: DMF) and dialysed with regenerated cellulose membranes in methanol. 1 H, 13 C and 23 Na NMR spectra were recorded in acetone- d 6 , DMSO- d 6 , and CDCl 2 at 30 °C on a JEOL JNM-LA500 spectrometer, operating at 500 ( 1 H), 125 ( 13 C) and 132 ( 23 Na) MHz, respectively. MALDI-TOF-MS analysis was performed on a Shimadzu AXIMA-CFR instrument equipped with 1.2 m linear flight tubes and a 337-nm nitrogen laser with dithranol (1,8,9-anthracenetriol) as an ionizing matrix and sodium trifluoroacetate as a cationizing agent. Electrospray ionization mass spectrometry was performed on Waters Quattro micro API. Dynamic light scattering was measured on Otsuka Photal ELSZ-0 equipped with a semiconductor laser (wavelength=658 nm) at 25 °C. The measuring angle was 165°, and the data was analysed by the CONTIN fitting method. Ultraviolet–visible spectra were obtained from Shimadzu UV-1,800 in H 2 O or CH 2 ClCH 2 Cl at r.t. (optical path length=1.0 cm). The cloud points of the polymers in water were determined by the transmittance of aqueous solution of polymers and monitored at 660 nm by changing the solution temperature between 20 and 80 °C (optical path length=1.0 cm; heating rate=1 °C min −1 ; cooling rate= −1 °C min −1 ) on Shimadzu UV-1800. How to cite this article: Terashima, T. et al . Polymeric pseudo-crown ether for cation recognition via cation template-assisted cyclopolymerization. Nat. Commun. 4:2321 doi: 10.1038/ncomms3321 (2013).